Arid5b facilitates chondrogenesis by recruiting the histone demethylase Phf2 to Sox9-regulated genes Histone modification, a critical step for epigenetic regulation, is an important modulator of biological events. Sox9 is a transcription factor critical for endochondral ossification; however, proof of its epigenetic regulation remains elusive. Here we identify AT-rich interactive domain 5b (Arid5b) as a transcriptional co-regulator of Sox9. Arid5b physically associates with Sox9 and synergistically induces chondrogenesis. Growth of Arid5b −/− mice is retarded with delayed endochondral ossification. Sox9-dependent chondrogenesis is attenuated in Arid5b-deficient cells. Arid5b recruits Phf2, a histone lysine demethylase, to the promoter region of Sox9 target genes and stimulates H3K9me2 demethylation of these genes. In the promoters of chondrogenic marker genes, H3K9me2 levels are increased in Arid5b −/− chondrocytes. Finally, we show that Phf2 knockdown inhibits Sox9-induced chondrocyte differentiation. Our findings establish an epigenomic mechanism of skeletal development, whereby Arid5b promotes chondrogenesis by facilitating Phf2-mediated histone demethylation of Sox9-regulated chondrogenic gene promoters. Skeletal development in vertebrates is mediated by two biological processes: intramembranous and endochondral ossification. Intramembranous ossification is used directly by osteoblasts, and occurs in the clavicle, cranial vault, some facial bones and parts of the mandible [1] . By contrast, endochondral ossification occurs in most bones including the ribs and long bones of the limbs, where a cartilaginous template is first developed in the embryo and is then replaced by a bone [2] . Endochondral ossification starts with mesenchymal cell condensation, and these cells undergo well-organized steps of chondrocyte differentiation. In the early stages of endochondral ossification, chondrocytes proliferate and vigorously produce chondrogenic extracellular matrix, composed of Col2a1, Col11a1 and Aggrecan, which drives skeletal growth and patterning [3] , [4] . Subsequently, these chondrocytes become pre-hypertrophic chondrocytes and further differentiate into hypertrophic chondrocytes that express Col10a1 (ref. 5 ). In the terminal stages, the chondrocyte matrix is mineralized, vascular vessels invade the calcified cartilage, and the cartilage is finally replaced by bone. These sequential steps are concomitantly regulated by various transcription factors in a spatial temporal manner. The transcription factor Sox9 (Sex determining region Y-type high-mobility group box protein 9) is the principal regulator of early chondrogenesis [3] , [4] . It promotes chondrocyte differentiation of mesenchymal stem cells by directly regulating chondrocyte matrix gene expression [6] , [7] . Sox9 also induces its transcriptional co-activators Sox5 and Sox6, and their transcriptional cooperation is important for successive chondrogenesis [6] , [8] . SOX9 haploinsufficiency in humans causes campomelic dysplasia characterized by severe chondrodysplasia [9] , [10] , and mutations around the SOX9 gene that disrupt SOX9 transcription cause Pierre Robin Sequence characterized by a cleft palate [11] . A critical role for Sox9 in chondrogenesis has also been demonstrated by genetic approaches in mice, where chondrocyte-specific Sox9 deficiency impairs endochondral ossification [12] , [13] . During transcription, DNA-binding transcription factors recruit transcriptional co-regulators as well as a set of basic transcription factors. Each component of this complex controls gene expression by regulating histone modification, chromatin remodelling, activation of basal transcription factors and mRNA splicing [14] . Thus, the identification and characterization of Sox9 transcriptional co-regulators is important for understanding the mechanism of chondrogenesis. Several Sox9 co-regulators, including CBP/p300, PGC-1α and Wwp2, have been identified [15] , [16] , [17] , and we previously used high-throughput assays to show that p54 nrb /NonO (ref. 18 ), which links Sox9-mediated transcription with RNA processing during chondrogenesis, and Znf219 (ref. 19 ) are members of the Sox9-assembled transcriptional complex. Histone modification is an essential process for transcription, and transcriptional co-regulators are prominently involved in this process [20] , [21] . There are eight types of histone modifications that have been identified, including acetylation, methylation and phosphorylation [21] . Of these, histone methylation/demethylation has emerged as an essential upstream signal for transcription, and the physiologic and pathologic significance of histone methylation/demethylation has been widely reported [22] , [23] . However, despite its importance in gene expression pathways, neither the molecular basis of histone methylation/demethylation during chondrogenesis nor its regulation by Sox9 transcriptional co-regulators has been fully elucidated. In this study, we identify Arid5b (AT-rich interactive domain 5B) as a transcriptional co-regulator for Sox9, and demonstrate that Arid5b is crucial for chondrogenesis both in vitro and in vivo . Furthermore, we show that Arid5b regulates the histone demethylation of Sox9 target gene promoters by recruiting the histone demethylase Phf2 to the promoter region. These results indicate that Arid5b is a critical transcriptional co-regulator for Sox9, and promotes chondrogenesis through histone modification. Our findings provide new insights into the epigenetic regulation of chondrogenic genes that are critical for endochondral ossification. Identification of Arid5b as a co-regulator for Sox9 To identify novel transcriptional co-regulators for Sox9 that are involved in chondrocyte differentiation, we took advantage of the notable difference between two fibroblastic cell lines, C3H10T1/2 and NIH-3T3, in their differentiation into chondrocytes. Similar levels of overexpressed Sox9 resulted in a marked increase in Col2a1 expression in C3H10T1/2 cells compared with NIH-3T3 cells ( Fig. 1a,b ). We reasoned that the high chondrocyte-differentiating activity of C3H10T1/2 cells arises from a greater expression of transcriptional co-regulators for Sox9 compared with those in NIH-3T3 cells. 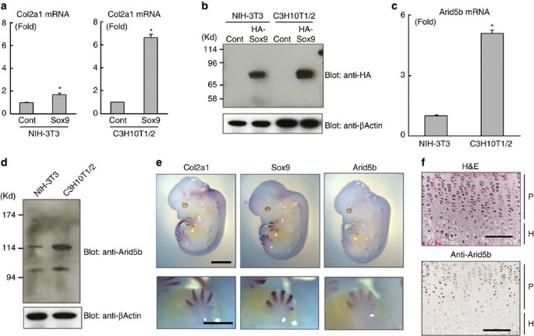Figure 1: Identification of Arid5b as a candidate transcriptional co-regulator for Sox9. (a) Effect of Sox9 onCol2a1expression in NIH-3T3 and C3H10T1/2 cells. NIH-3T3 (left) and C3H10T1/2 cells (right) were infected with control (Cont) or Sox9 adenovirus at 20 MOI and cultured for 4 days. Total RNA was isolated and subjected to real-time PCR. Data are shown as the mean±s.d. (n=3) *P<0.01 (versus Cont); Student’st-test. (b) NIH-3T3 (left) and C3H10T1/2 cells (right) were infected with control (Cont) or HA-Sox9 adenovirus and cultured for 4 days. Cell lysates were analysed using immunoblotting with anti-HA and anti-β-actin antibodies. Sox9 expression was similar in NIH-3T3 and C3H10T1/2 cells. (c) Expression ofArid5bmRNA in NIH-3T3 and C3H10T1/2 cells. Total RNA was isolated from 80% confluent NIH-3T3 and C3H10T1/2 cells and analysed by real-time PCR. Data are shown as the mean±s.d. (n=3). *P<0.01 (versus NIH-3T3); Student’st-test. (d) Expression of endogenous Arid5b in NIH-3T3 and C3H10T1/2 cells. Cell lysates were isolated from NIH-3T3 and C3H10T1/2 cells and analysed using immunoblotting with an anti-Arid5b antibody. β-actin was used as a loading control. Bands representing both the longer and shorter splice variants of Arid5b are visible. (e) Expression of Arid5b in developing limb buds. The expression ofArid5b,Col2a1andSox9was similar in developing limbs in E12.5 mice, as determined by whole-mountin situhybridization. Scale bar, 2 mm (upper panel), 1 mm (lower panel). (f) Immunohistochemical analysis of Arid5b in growth plate chondrocytes. Paraffin sections of a 3-week-old mouse tibia were subjected to H&E staining (upper panel) and immunocytochemical analyses using anti-Arid5b antibody (lower panel). Scale bar, 100 μm. H, hypertrophic chondrocytes; P, proliferating chondrocytes. Based on this, we performed gene expression profiling using Solexa deep sequencing technology, and selected transcription factors that showed higher expression in C3H10T1/2 cells ( Table 1 ). Among the top 10 candidate genes, we focused on Arid5b because its involvement in chondrogenesis had not yet been examined. Arid5b belongs to the AT-rich interaction domain (ARID) family, which is defined by the presence of the helix-turn-helix motif-based ARID DNA-binding domain [24] . High expression of Arid5b in C3H10T1/2 cells was observed at both the mRNA and protein levels ( Fig. 1c,d ). Figure 1: Identification of Arid5b as a candidate transcriptional co-regulator for Sox9. ( a ) Effect of Sox9 on Col2a1 expression in NIH-3T3 and C3H10T1/2 cells. NIH-3T3 (left) and C3H10T1/2 cells (right) were infected with control (Cont) or Sox9 adenovirus at 20 MOI and cultured for 4 days. Total RNA was isolated and subjected to real-time PCR. Data are shown as the mean±s.d. ( n =3) * P <0.01 (versus Cont); Student’s t- test. ( b ) NIH-3T3 (left) and C3H10T1/2 cells (right) were infected with control (Cont) or HA-Sox9 adenovirus and cultured for 4 days. Cell lysates were analysed using immunoblotting with anti-HA and anti-β-actin antibodies. Sox9 expression was similar in NIH-3T3 and C3H10T1/2 cells. ( c ) Expression of Arid5b mRNA in NIH-3T3 and C3H10T1/2 cells. Total RNA was isolated from 80% confluent NIH-3T3 and C3H10T1/2 cells and analysed by real-time PCR. Data are shown as the mean±s.d. ( n= 3). * P <0.01 (versus NIH-3T3); Student’s t- test. ( d ) Expression of endogenous Arid5b in NIH-3T3 and C3H10T1/2 cells. Cell lysates were isolated from NIH-3T3 and C3H10T1/2 cells and analysed using immunoblotting with an anti-Arid5b antibody. β-actin was used as a loading control. Bands representing both the longer and shorter splice variants of Arid5b are visible. ( e ) Expression of Arid5b in developing limb buds. The expression of Arid5b , Col2a1 and Sox9 was similar in developing limbs in E12.5 mice, as determined by whole-mount in situ hybridization. Scale bar, 2 mm (upper panel), 1 mm (lower panel). ( f ) Immunohistochemical analysis of Arid5b in growth plate chondrocytes. Paraffin sections of a 3-week-old mouse tibia were subjected to H&E staining (upper panel) and immunocytochemical analyses using anti-Arid5b antibody (lower panel). Scale bar, 100 μm. H, hypertrophic chondrocytes; P, proliferating chondrocytes. Full size image Table 1 Top 10 highly tagged genes in C3H10T1/2 cells expressed more than two-fold higher than in NIH-3T3 cells. Full size table To test whether Arid5b was involved in chondrocyte differentiation, we first examined its expression in cartilage. Whole-mount in situ hybridization demonstrated clear co-expression of Col2a1 , Sox9 and Arid5b mRNA in the developing limbs ( Fig. 1e ). Time course analysis of Arid5b expression in insulin-treated ATDC5, a chondrogenic cell line, demonstrated a parallel increase of Arid5b with Sox9 , Col2a1 and Aggrecan during chondrocyte differentiation ( Supplementary Fig. S1 ). Of note, Arid5b was specifically expressed in proliferating growth plate chondrocytes as determined by immunohistochemical analysis ( Fig. 1f ). Although Arid5b was expressed in Sertoli cells in the testis, where Sox9 also has an important role, its expression pattern differed from that of Sox9 ( Supplementary Fig. S2 ). Collectively, these data suggest that Arid5b has a unique and specific role in chondrocyte differentiation. Arid5b promotes chondrogenesis by stimulating Sox9 function We next determined the functional role of Arid5b in chondrocyte differentiation. Although the overexpression of Arid5b alone increased Col2a1 expression in C3H10T1/2 cells, the concomitant overexpression of Arid5b and Sox9 synergistically increased the expression levels of Col2a1 and Aggrecan ( Fig. 2a ). Functional cooperation between Arid5b and Sox9 was also observed at the transcriptional level, as assessed by reporter assays using a Col2a1 promoter construct containing four repeats of Sox9-binding elements present in intron 1 of the Col2a1 gene ( Fig. 2b ). It should be noted that introduction of Arid5b in NIH-3T3 cells increased Sox9-induced Col2a1 expression ( Fig. 2c ). By contrast, Arid5b overexpression alone in either cell line failed to induce Sox9 expression, and Sox9 alone or Sox9 together with Sox5 and Sox6 did not affect Arid5b expression ( Supplementary Fig. S3a,b ). 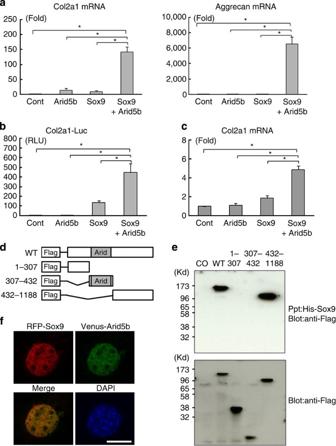Figure 2: Stimulation of Sox9-dependent chondrocyte differentiation by Arid5b. (a) C3H10T1/2 cells were infected with control (Cont), Arid5b, Sox9 or both Arid5b and Sox9 adenoviruses and then cultured for 4 days. Total RNA was analysed by real-time PCR forCol2a1andAggrecan. Data are shown as the mean±s.d. (n=3). *P<0.01; one-way ANOVA followed by the Tukey–Kramer test. (b) C3H10T1/2 cells were transfected with a Col2a1–luciferase construct (Col2a1-Luc) together with an empty vector (pcDNA3, Cont), Arid5b, Sox9 or both Arid5b and Sox9. Luciferase activities were measured 48 h after transfection. Data are expressed in relative luciferase units (mean±s.d.,n=3). *P<0.01; one-way ANOVA followed by the Tukey–Kramer test. (c) NIH-3T3 cells were infected with control (Cont), Arid5b, Sox9 or both Arid5b and Sox9 adenoviruses and then cultured for 4 days.Col2a1andAggrecanmRNA levels were determined by real-time PCR. Data are shown as the mean±s.d. (n=3). *P<0.01; one-way ANOVA followed by the Tukey–Kramer test. (d) Schematic diagram of the Arid5b deletion mutants. The ARID DNA-binding domain is depicted as a grey bar. (e) Arid5b physically interacts with Sox9. 293FT cells were transfected with 3 × Flag-tagged WT or Arid5b mutants. Cell lysates were precipitated with His-tagged Sox9 and analysed by immunoblotting with an anti-Flag antibody (upper panel, precipitated Arid5b; lower panel, cell lysates). (f) Colocalization of Arid5b and Sox9 in the nucleus. C3H10T1/2 cells transfected with Venus-tagged Arid5b (Venus-Arid5b) and RFP-tagged Sox9 (RFP-Sox9) were visualized under a fluorescence microscope (original magnification, × 63). Scale bar, 10 μm. Figure 2: Stimulation of Sox9-dependent chondrocyte differentiation by Arid5b. ( a ) C3H10T1/2 cells were infected with control (Cont), Arid5b, Sox9 or both Arid5b and Sox9 adenoviruses and then cultured for 4 days. Total RNA was analysed by real-time PCR for Col2a1 and Aggrecan . Data are shown as the mean±s.d. ( n =3). * P <0.01; one-way ANOVA followed by the Tukey–Kramer test. ( b ) C3H10T1/2 cells were transfected with a Col2a1–luciferase construct (Col2a1-Luc) together with an empty vector (pcDNA3, Cont), Arid5b, Sox9 or both Arid5b and Sox9. Luciferase activities were measured 48 h after transfection. Data are expressed in relative luciferase units (mean±s.d., n =3). * P <0.01; one-way ANOVA followed by the Tukey–Kramer test. ( c ) NIH-3T3 cells were infected with control (Cont), Arid5b, Sox9 or both Arid5b and Sox9 adenoviruses and then cultured for 4 days. Col2a1 and Aggrecan mRNA levels were determined by real-time PCR. Data are shown as the mean±s.d. ( n =3). * P <0.01; one-way ANOVA followed by the Tukey–Kramer test. ( d ) Schematic diagram of the Arid5b deletion mutants. The ARID DNA-binding domain is depicted as a grey bar. ( e ) Arid5b physically interacts with Sox9. 293FT cells were transfected with 3 × Flag-tagged WT or Arid5b mutants. Cell lysates were precipitated with His-tagged Sox9 and analysed by immunoblotting with an anti-Flag antibody (upper panel, precipitated Arid5b; lower panel, cell lysates). ( f ) Colocalization of Arid5b and Sox9 in the nucleus. C3H10T1/2 cells transfected with Venus-tagged Arid5b (Venus-Arid5b) and RFP-tagged Sox9 (RFP-Sox9) were visualized under a fluorescence microscope (original magnification, × 63). Scale bar, 10 μm. Full size image We next tested whether Arid5b could physically associate with Sox9 using in vitro binding assays with a series of deletion mutants of Arid5b ( Fig. 2d ). Arid5b physically interacted with Sox9 by means of the C terminus of Arid5b ( Fig. 2e ). Moreover, Venus-tagged Arid5b colocalized with RFP-tagged Sox9 in the nucleus ( Fig. 2f ). To further investigate the functional role of Arid5b in chondrocyte differentiation, we tested whether Arid5b directly controls Col2a1 expression. We found that the Col2a1 promoter contains a putative Arid5b-binding sequence motif, which almost fits the core consensus sequence ( Fig. 3a ) [25] . Chromatin immunoprecipitation (ChIP) assays and DNA pull-down assays using the biotinylated Arid5b-binding element revealed that Arid5b directly bound this element ( Fig. 3b–d ). Moreover, direct binding of Arid5b to the Arid5b-binding element was strongly competed with by excess non-biotinylated probe ( Fig. 3d ). Finally, we found that functional cooperation between Sox9 and Arid5b was markedly attenuated by the introduction of a mutated Arid5b-binding element in the Col2a1 promoter (catat→ TG tat) ( Fig. 3e ). In addition to the Col2a1 promoter, ChIP assays also demonstrated that Arid5b could directly bind to the Arid5b-binding sequence in the Aggrecan promoter ( Supplementary Fig. S4 ). Taken together, these results suggest that Arid5b promotes the expression of genes involved in chondrocyte differentiation as a transcriptional co-regulator for Sox9. 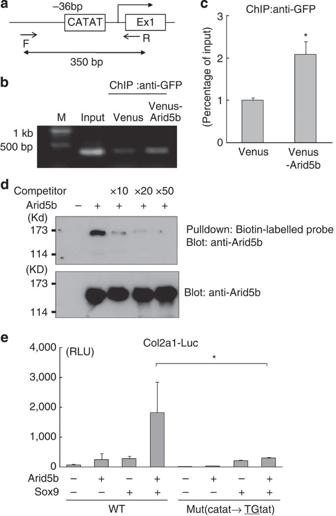Figure 3: Arid5b directly regulates Col2a1 expression. (a) Schematic presentation of the putative Arid5b-binding element (CATAT) and primers used for ChIP assays in the promoter region of mouseCol2a1. (b,c) ChIP assays. C3H10T1/2 cells were infected with Venus or Venus-Arid5b adenovirus and then immunoprecipitated with anti-GFP antibodies. The binding of Arid5b to theCol2a1promoter region was examined by PCR using the primers shown in (a). The binding of Arid5b to theCol2a1promoter region was also examined by real-time PCR. Data are shown as percentages of input (mean±s.d.,n=3) *P<0.01 (versus Venus); Student’st-test. (d) DNA pull-down assays using the Arid5b-binding element in theCol2a1promoter. Lysates of 293FT cells transfected with empty or Flag-Arid5b vector were incubated with biotinylated oligonucleotide containing a putative Arid5b-binding element in theCol2a1promoter in the presence or absence of the unlabelled oligonucleotide (competitor). After precipitation with streptavidin beads, proteins associated with the oligonucleotide were determined by immunoblotting with an anti-Arid5b antibody. (e) Mutation analysis of the Arid5b-binding element in theCol2a1promoter. C3H10T1/2 cells were transfected with a WT or mutantCol2a1–luciferase construct together with the indicated expression vectors. Luciferase activities were measured 48 h after transfection. Data are expressed in relative luciferase units (mean±s.d.,n=3). *P<0.01; two-way ANOVA followed by a Tukey’s HSDpost hoctest. Figure 3: Arid5b directly regulates Col2a1 expression. ( a ) Schematic presentation of the putative Arid5b-binding element (CATAT) and primers used for ChIP assays in the promoter region of mouse Col2a1 . ( b , c ) ChIP assays. C3H10T1/2 cells were infected with Venus or Venus-Arid5b adenovirus and then immunoprecipitated with anti-GFP antibodies. The binding of Arid5b to the Col2a1 promoter region was examined by PCR using the primers shown in ( a ). The binding of Arid5b to the Col2a1 promoter region was also examined by real-time PCR. Data are shown as percentages of input (mean±s.d., n =3) * P <0.01 (versus Venus); Student’s t- test. ( d ) DNA pull-down assays using the Arid5b-binding element in the Col2a1 promoter. Lysates of 293FT cells transfected with empty or Flag-Arid5b vector were incubated with biotinylated oligonucleotide containing a putative Arid5b-binding element in the Col2a1 promoter in the presence or absence of the unlabelled oligonucleotide (competitor). After precipitation with streptavidin beads, proteins associated with the oligonucleotide were determined by immunoblotting with an anti-Arid5b antibody. ( e ) Mutation analysis of the Arid5b-binding element in the Col2a1 promoter. C3H10T1/2 cells were transfected with a WT or mutant Col2a1 –luciferase construct together with the indicated expression vectors. Luciferase activities were measured 48 h after transfection. Data are expressed in relative luciferase units (mean±s.d., n =3). * P <0.01; two-way ANOVA followed by a Tukey’s HSD post hoc test. Full size image Arid5b is critical for endochondral ossification in vivo We next used Arid5b-deficient mice to examine whether Arid5b regulates endochondral ossification in vivo [26] . Analysis of 3-week-old mice revealed that Arid5b −/− mice exhibited a dwarf phenotype compared with wild-type (WT) mice ( Supplementary Fig. S5a ). Histological examination of tibial growth plate chondrocytes demonstrated that Arid5b −/− mice showed a marked reduction in the width of the Col2-positive area ( Fig. 4a and Supplementary Fig. S5b ). This suggested that Arid5b was important for postnatal skeletal development. Moreover, even at P0, Arid5b −/− mice showed a dwarf phenotype with shortened tibia length compared with WT mice ( Supplementary Fig. S5c ). 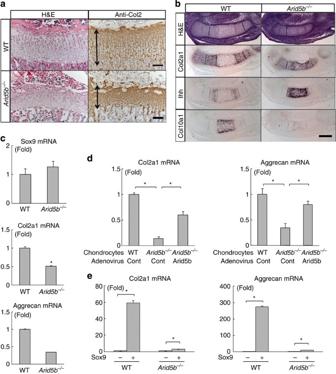Figure 4:Delayed endochondral ossification with impaired early chondrogenesis inArid5b−/−mice. (a) Immunohistochemical analysis of tibial growth plate chondrocytes in 3-week-old WT andArid5b−/−mice. Paraffin sections of tibias from 3-week-old littermates were subjected to immunocytochemical analyses using an anti-Col2 antibody. Scale bar, 100 μm. The width of the Col2-positive area was shortened inArid5b−/−mice compared with WT mice. (b) Sections of tibia from E14.5 WT andArid5b−/−littermate embryos were examined by H&E staining andin situhybridization using antisense probes againstCol2a1,IhhorCol10a1. Scale bar, 200 μm. (c) Total RNA was isolated from the hindlimbs of E14.5 WT andArid5b−/−littermate embryos and mRNA expression ofSox9,Col2a1andAggrecanwas determined by real-time PCR. Data are shown as fold expression normalized to WT (mean±s.d.,n=3). *P<0.01 (versus WT); Student’st-test. (d) Primary chondrocytes from WT andArid5b−/−littermate mice were infected with control (Cont) or Arid5b adenovirus and cultured for 4 days. Total RNA was isolated and mRNA expression ofCol2a1andAggrecanwas determined by real-time PCR. Data are shown as the mean±s.d. (n=3) *P<0.01; one-way ANOVA followed by the Tukey–Kramer test. (e) Primary chondrocytes from WT andArid5b−/−littermate mice were infected with control (Cont) or Sox9 adenovirus and cultured for 4 days. Total RNA was isolated and mRNA expression ofCol2a1andAggrecanwas determined by real-time PCR. Data are shown as the mean±s.d. (n=3). *P<0.01 (versus Sox9(−)); Student’st-test. Figure 4: Delayed endochondral ossification with impaired early chondrogenesis in Arid5b −/− mice. ( a ) Immunohistochemical analysis of tibial growth plate chondrocytes in 3-week-old WT and Arid5b −/− mice. Paraffin sections of tibias from 3-week-old littermates were subjected to immunocytochemical analyses using an anti-Col2 antibody. Scale bar, 100 μm. The width of the Col2-positive area was shortened in Arid5b −/− mice compared with WT mice. ( b ) Sections of tibia from E14.5 WT and Arid5b −/− littermate embryos were examined by H&E staining and in situ hybridization using antisense probes against Col2a1 , Ihh or Col10a1 . Scale bar, 200 μm. ( c ) Total RNA was isolated from the hindlimbs of E14.5 WT and Arid5b −/− littermate embryos and mRNA expression of Sox9 , Col2a1 and Aggrecan was determined by real-time PCR. Data are shown as fold expression normalized to WT (mean±s.d., n =3). * P <0.01 (versus WT); Student’s t- test. ( d ) Primary chondrocytes from WT and Arid5b −/− littermate mice were infected with control (Cont) or Arid5b adenovirus and cultured for 4 days. Total RNA was isolated and mRNA expression of Col2a1 and Aggrecan was determined by real-time PCR. Data are shown as the mean±s.d. ( n =3) * P <0.01; one-way ANOVA followed by the Tukey–Kramer test. ( e ) Primary chondrocytes from WT and Arid5b −/− littermate mice were infected with control (Cont) or Sox9 adenovirus and cultured for 4 days. Total RNA was isolated and mRNA expression of Col2a1 and Aggrecan was determined by real-time PCR. Data are shown as the mean±s.d. ( n =3). * P <0.01 (versus Sox9(−)); Student’s t- test. Full size image To further clarify the in vivo significance of Arid5b in endochondral ossification, we examined the fetal growth plate of the tibia by in situ hybridization analysis. E14.5 Arid5b −/− mice showed a slightly dwarf phenotype compared with WT mice ( Supplementary Fig. S5d ). Histological analysis revealed that the Col2a1 -positive zone of tibias from E14.5 Arid5b −/− mice was not separated by Indian hedgehog ( Ihh )-positive chondrocytes ( Fig. 4b ). Moreover, Ihh -positive chondrocytes were diffusely expressed, and a Col10 -positive hypertrophic zone was not detected in the tibias of Arid5b −/− mice ( Fig. 4b ). In situ hybridization analysis using tibias from E18.5 mice demonstrated a marginal impairment of endochondral ossification compared with that in E14.5 Arid5b −/− mice ( Supplementary Fig. S6 ). These data suggested that the delay in endochondral ossification shown in Arid5b −/− mice was likely a result of impaired early-stage chondrocyte differentiation. Analysis of mRNA isolated from the hindlimbs of WT and Arid5b −/− mice revealed that the expression of Col2a1 and Aggrecan mRNA was decreased in Arid5b −/− mice compared with WT mice, whereas the expression of Sox9 was not affected ( Fig. 4c ). Collectively, these results imply that chondrocyte differentiation in the Sox9-regulated stage was attenuated in Arid5b −/− mice, and consequently delayed endochondral ossification. To further examine the biological role of Arid5b in chondrocyte differentiation, we assessed the differentiating activity of primary chondrocytes isolated from P0 rib cartilage of WT and Arid5b −/− mice. Col2a1 and Aggrecan mRNA expression was markedly decreased in primary chondrocytes isolated from Arid5b −/− mice ( Fig. 4d ). Importantly, the decreased chondrocyte marker gene expression in Arid5b −/− mice was restored by infection of Arid5b adenovirus ( Fig. 4d ). BMP2-induced chondrocyte differentiation, assessed by Alcian Blue positive matrix accumulation, was also attenuated in Arid5b −/− chondrocytes ( Supplementary Fig. S7a ). Induction of Col2a1 and Aggrecan mRNA by BMP2 was substantially suppressed in primary chondrocytes isolated from Arid5b −/− mice ( Supplementary Fig. S7b ). Furthermore, Sox9-dependent Col2a1 and Aggrecan expression was markedly reduced in chondrocytes of Arid5b −/− compared with WT mice ( Fig. 4e ). Taken together, these results suggest that Arid5b is a critical co-regulator for Sox9-dependent chondrocyte differentiation in vivo and is essential for the subsequent endochondral ossification steps. Arid5b mutant inhibits chondrogenesis To gain further insight into the role of Arid5b in chondrogenesis, we evaluated the effect of overexpressing Arid5b deletion mutants on endochondral ossification. An Arid5b (307–432) mutant, which contains only an ARID domain and lacks the ability to interact with Sox9, suppressed the transcriptional activity of Sox9 on the Col2a1 promoter ( Supplementary Fig. S8a ). In addition, overexpression of this mutant inhibited Col2a1 expression induced by Sox9 and Sox5/6/9 ( Supplementary Fig. S8b ). Moreover, this mutant inhibited chondrocyte differentiation of limb bud cells in a micromass culture system, as determined by Alcian Blue staining, and decreased Col2a1 and Aggrecan expression induced by BMP2 ( Supplementary Fig. S8c ). These results collectively indicate that Arid5b (307–432), which can bind to the Arid5b-binding element but cannot interact with Sox9, has dominant negative effects on chondrocyte differentiation. To further evaluate the dominant inhibitory effect of Arid5b (307–432) on endochondral ossification, we generated transgenic (Tg) mice that overexpress this mutant during the mesenchymal condensation stage under the control of the Prx-1 gene promoter ( Supplementary Fig. S8d ). IRES–EGFP was integrated in the transgenic construct to follow transgene expression, which was confirmed by fluorescence stereomicroscopy ( Supplementary Fig. S8e ). Immunohistochemical analysis using E14.5 mice tibia demonstrated that the Col2-positive zone was shortened in Tg mice ( Supplementary Fig. S8f ). Moreover, Col2a1 and Aggrecan mRNA expression isolated from E14.5 Tg hindlimbs was decreased compared with WT mice ( Supplementary Fig. S8g ). Thus, these results suggest that the Arid5b (307–432) mutant negatively regulates cartilage development in vitro and in vivo . Arid5b controls H3K9me2 of Sox9 target promoters via Phf2 We next investigated the precise molecular mechanism by which Arid5b regulates endochondral ossification as a co-regulator of Sox9. Recent findings indicated that Arid5b forms a transcriptional complex with Phf2, a jmjC histone lysine demethylase, through an N-terminal region and promotes the demethylation of dimethylated Lys 9 on histone H3 (H3K9me2) [27] . We observed a physical interaction between Arid5b and Phf2 using co-immunoprecipitation analysis ( Fig. 5a ) and a pull-down assay ( Supplementary Fig. S9 ). As the biological significance of Arid5b and Phf2 interaction has not been studied, we attempted to examine whether the interaction between Arid5b and Phf2 is involved in regulating chondrogenesis. H3K9me2 is the repressive histone methylation mark of gene transcription, and H3K9me2 demethylation of target gene promoters by histone lysine demethylases permits transcription [27] . Thus, we hypothesized that Arid5b and Phf2 complexes modulate H3K9me2 levels of chondrocyte marker gene promoters and subsequently allow Sox9-induced chondrogenic gene transcription. To test this, we first determined whether Arid5b recruits Phf2 to the Col2a1 promoter region by ChIP assays using a Phf2 antibody. Although overexpression of Arid5b did not change Phf2 mRNA or protein levels ( Fig. 5b,c ), it did increase the association between Phf2 and the promoters of Col2a1 and Aggrecan ( Fig. 5d , Supplementary Fig. S10a ). Accordingly, the levels of H3K9me2 in the Col2a1 promoter were markedly decreased by Arid5b overexpression ( Fig. 5e ). By contrast, Arid5b had no effect on the H3K9me2 status of the promoter regions of Col1a1 , an osteoblast marker gene, and Myogenin , a myoblast marker gene, in C3H10T1/2 cells ( Fig. 5e ). These data suggest that Arid5b recruits Phf2 to the Col2a1 promoter and promotes the demethylation of H3K9me2 specifically in this promoter. 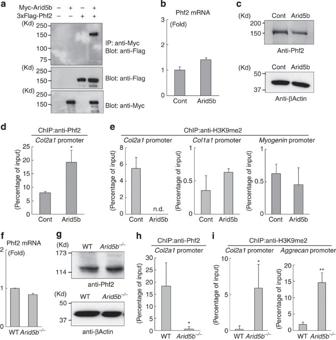Figure 5:Arid5b recruits Phf2 to theCol2a1promoter and leads to H3K9me2 demethylation. (a) Myc-Arid5b and Flag-Phf2 were transfected into 293FT cells and incubated for 48 h. Cell lysates were immunoprecipitated with an anti-Myc antibody and immunoblotted with an anti-Flag antibody (top). The expression levels of Flag-Phf2 and Myc-Arid5b were monitored by immunoblotting with an anti-Flag (middle) or anti-Myc (bottom) antibody. (b,c) C3H10T1/2 cells were infected with Arid5b adenovirus, and the expression of Phf2 was evaluated by real-time PCR (mean±s.d.,n=3) (b) and immunoblotting with an anti-Phf2 antibody (c, upper panel). β-actin was used as a loading control (c, lower panel). (d) Arid5b was overexpressed in C3H10T1/2 cells and ChIP assays were conducted using an anti-Phf2 antibody. Data are shown as percentages of input (mean±s.d.,n=3). *P<0.05 (versus Cont); Student’st-test. (e) Arid5b was overexpressed in C3H10T1/2 cells and the levels of H3K9me2 were examined by ChIP assays using an anti-H3K9me2 antibody. Data are shown as percentages of input (mean±s.d.,n=3). n.d.: not detectable. (f,g) Expression of Phf2 in primary chondrocytes isolated from newborn WT andArid5b−/−mice. The expression of Phf2 mRNA was evaluated by real-time PCR (f; mean±s.d.,n=3) and protein by immunoblotting with an anti-Phf2 antibody (g, upper panel). β-actin was used as a loading control (g, lower panel). (h) ChIP assays were performed using an anti-Phf2 antibody. Data are shown as percentages of input (mean±s.d.,n=3). *P<0.05 (versus Cont); Student’st-test. (i) The levels of H3K9me2 in WT andArid5b−/−chondrocytes were examined by ChIP assays using an anti-H3K9me2 antibody. Data are shown as percentages of input (mean±s.d.,n=3). **P<0.01, *P<0.05 (versus WT); Student’st-test. Figure 5: Arid5b recruits Phf2 to the Col2a1 promoter and leads to H3K9me2 demethylation. ( a ) Myc-Arid5b and Flag-Phf2 were transfected into 293FT cells and incubated for 48 h. Cell lysates were immunoprecipitated with an anti-Myc antibody and immunoblotted with an anti-Flag antibody (top). The expression levels of Flag-Phf2 and Myc-Arid5b were monitored by immunoblotting with an anti-Flag (middle) or anti-Myc (bottom) antibody. ( b , c ) C3H10T1/2 cells were infected with Arid5b adenovirus, and the expression of Phf2 was evaluated by real-time PCR (mean±s.d., n =3) ( b ) and immunoblotting with an anti-Phf2 antibody ( c , upper panel). β-actin was used as a loading control ( c , lower panel). ( d ) Arid5b was overexpressed in C3H10T1/2 cells and ChIP assays were conducted using an anti-Phf2 antibody. Data are shown as percentages of input (mean±s.d., n =3). * P <0.05 (versus Cont); Student’s t- test. ( e ) Arid5b was overexpressed in C3H10T1/2 cells and the levels of H3K9me2 were examined by ChIP assays using an anti-H3K9me2 antibody. Data are shown as percentages of input (mean±s.d., n =3). n.d.: not detectable. ( f , g ) Expression of Phf2 in primary chondrocytes isolated from newborn WT and Arid5b −/− mice. The expression of Phf2 mRNA was evaluated by real-time PCR (f; mean±s.d., n =3) and protein by immunoblotting with an anti-Phf2 antibody ( g , upper panel). β-actin was used as a loading control ( g , lower panel). ( h ) ChIP assays were performed using an anti-Phf2 antibody. Data are shown as percentages of input (mean±s.d., n =3). * P <0.05 (versus Cont); Student’s t -test. ( i ) The levels of H3K9me2 in WT and Arid5b −/− chondrocytes were examined by ChIP assays using an anti-H3K9me2 antibody. Data are shown as percentages of input (mean±s.d., n =3). ** P <0.01, * P <0.05 (versus WT); Student’s t- test. Full size image To further understand the relationship between Arid5b and Phf2 during chondrogenesis, we examined the H3K9me2 levels of chondrogenic gene promoters in primary chondrocytes isolated from Arid5b −/− mice. Although WT and Arid5b −/− chondrocytes were found to express similar levels of Phf2 ( Fig. 5f,g ), the interaction between Phf2 and the promoter of Col2a1 was reduced in Arid5b −/− chondrocytes ( Fig. 5h ). Similarly, the recruitment of Phf2 to the Aggrecan promoter was decreased in Arid5b −/− chondrocytes ( Supplementary Fig. S10b ). In contrast to the effect of Arid5b overexpression on H3K9me2 levels ( Fig. 5e ), H3K9me2 levels of the Col2a1 and Aggrecan promoters were markedly increased in primary chondrocytes isolated from Arid5b −/− mice ( Fig. 5i ). There were no significant differences in the recruitment of Phf2 to the promoters of Col1a1 and Myogenin in WT and Arid5b −/− mice; however, H3K9me2 levels of these promoters were increased in Arid5b −/− chondrocytes ( Supplementary Fig. S11 ). Together, these results suggest that Arid5b recruited Phf2 specifically to chondrogenic gene promoters to promote H3K9me2 demethylation, thereby removing the repression of chondrogenic gene transcription. Previous studies have indicated that Arid5a also promotes chondrogenesis cooperatively with Sox9 (ref. 28 ). Therefore, we hypothesized that Arid5a may also interact with Phf2 to stimulate chondrogenesis. To examine whether Arid5a could cooperate with Phf2, we performed pull-down assays using the N-terminal region, which is responsible for the association between Arid5 family members and Phf2 ( Supplementary Fig. S9a ) [27] . We were unable to detect any physical interaction between Phf2 and Arid5a ( Supplementary Fig. S9b ). Furthermore, Arid5a could not restore the reduction of Col2a1 and Aggrecan expression observed in Arid5b −/− chondrocytes ( Supplementary Fig. S12 ). This suggests that Arid5a does not cooperate with Phf2 during chondrogenesis, and instead regulates chondrogenesis by a different mechanism [28] . Finally, we tested whether Phf2 is involved in Sox9-induced chondrogenic gene expression. To this end, we knocked down Phf2 expression by siRNA in primary chondrocytes and monitored chondrogenic gene expression ( Fig. 6a ). Although the knockdown of Phf2 had no effect on Sox9 and Arid5b expression, Col2a1 expression was slightly decreased ( Fig. 6b ). Of interest, the knockdown of Phf2 decreased Sox9-induced Col2a1 and Aggrecan mRNA expression ( Fig. 6b ), but did not affect Arid5b binding to the Col2a1 promoter ( Supplementary Fig. S13 ). These data suggest that Phf2-dependent H3K9me2 demethylation at Sox9-dependent promoters is a crucial step for endochondral ossification regulated by Sox9. 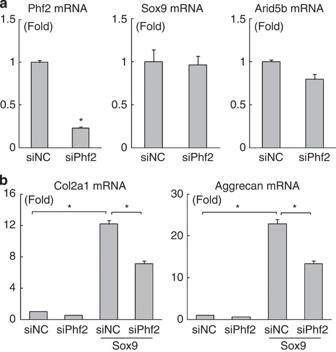Figure 6: Inhibition of Sox9-dependent chondrocyte differentiation by knockdown of Phf2. (a) Knockdown of Phf2 in primary chondrocytes by siRNA (siPhf2). Primary chondrocytes were transfected with Phf2 siRNA and non-targeted siRNA as a control (siNC). The expression ofPhf2,Sox9andArid5bwas examined by real-time PCR. Data are shown as fold expression normalized to siNC (mean±s.d.,n=3). *P<0.01 (versus siNC); Student’st-test. (b) Inhibition of chondrocyte differentiation by Phf2 siRNA. Primary chondrocytes transfected with siPhf2 or siNC were infected with Sox9 adenovirus. The expression ofCol2a1andAggrecanmRNA was determined by real-time PCR. Data are shown as fold expression normalized to siNC (mean±s.d.,n=3). *P<0.01; one-way ANOVA followed by the Tukey–Kramer test. Figure 6: Inhibition of Sox9-dependent chondrocyte differentiation by knockdown of Phf2. ( a ) Knockdown of Phf2 in primary chondrocytes by siRNA (siPhf2). Primary chondrocytes were transfected with Phf2 siRNA and non-targeted siRNA as a control (siNC). The expression of Phf2 , Sox9 and Arid5b was examined by real-time PCR. Data are shown as fold expression normalized to siNC (mean±s.d., n =3). * P <0.01 (versus siNC); Student’s t- test. ( b ) Inhibition of chondrocyte differentiation by Phf2 siRNA. Primary chondrocytes transfected with siPhf2 or siNC were infected with Sox9 adenovirus. The expression of Col2a1 and Aggrecan mRNA was determined by real-time PCR. Data are shown as fold expression normalized to siNC (mean±s.d., n =3). * P <0.01; one-way ANOVA followed by the Tukey–Kramer test. Full size image Transcriptional regulation involves dynamic protein–protein interactions between transcription factors and transcriptional co-regulators. These complexes coordinate the control of gene expression by histone modification, chromatin remodelling and mRNA splicing in a spatiotemporal manner [3] . Thus, the identification and characterization of novel co-regulators is important for a better understanding of the molecular basis of gene expression. Accumulating evidence indicates that many transcriptional regulators primarily affect epigenetic control, such as histone modification and chromatin remodelling. Although a variety of Sox9 co-regulators have been identified and characterized [15] , [16] , [17] , [18] , [28] , [29] , [30] , [31] , [32] , the co-regulators involved in the epigenetic regulation of chondrogenesis have yet to be fully elucidated. In this study, we identified Arid5b as a Sox9 co-regulator by gene expression profiling between different chondrogenic cell lines. We found that Arid5b promotes chondrogenesis cooperatively with Sox9 by recruiting the histone demethylase Phf2 to chondrogenic gene promoters and promoting subsequent histone demethylation ( Supplementary Fig. S14 ). Importantly, the discovery of the linkage between Arid5b/Phf2 and Sox9 indicates a tissue- and gene-specific role of the Arid5b/Phf2 complex in chondrogenesis, as well as a biological significance of this complex. Thus, our findings provide novel insights into the epigenetic regulation of chondrogenesis. We performed gene expression profiling using Solexa deep sequencing technology and identified Arid5b as a novel transcriptional co-regulator for Sox9. As digital quantification of gene expression by Solexa sequencing is much more precise than microarray analysis, our approach is valid for the identification of low abundance transcripts such as transcription factors. For example, NonO, which has a critical role in the mRNA splicing of Sox9 target genes [18] was also detected as a candidate gene by this process. Further analysis of candidate genes that are highly expressed in C3H10T1/2 cells may lead to the identification of novel and critical Sox9 transcriptional co-regulators involved in chondrogenesis. This is particularly relevant given our observation that the phenotype of Arid5b −/− mice is less severe than that of Sox9 −/− mice [12] , which suggests that unknown Sox9 co-regulators are likely to compensate for Arid5b function. Thus, the identification and characterization of Sox9 co-regulators will be important for improving our understanding of genetic regulation chondrogenesis. Arid5b was first cloned as a protein that bound to the transcriptional modulator region of the human cytomegalovirus major immediate-early promoter, and belongs to the ARID protein family [24] , [33] . The Arid domain is highly conserved in yeast (Swi1), drosophila (Dri) and mammals (p270, Bright and Jumonji), but family members have diverse functions, including cell growth, differentiation and development [33] . Although the biochemical functions of Arid5b are well studied in terms of DNA-binding activity and three-dimensional (3D) structure [25] , [34] , little is known about the cellular and biological functions of Arid5b. Structurally, Arid5b differs from other ARID proteins in several important aspects and therefore is predicted to have distinct functions. First, the ARID domain of Arid5b contains six helices, whereas p270, which is an integral member of the human SWI/SNF complex, contains eight helices [33] . Second, the amino acid sequences outside the ARID domain in Arid5b are not similar to those of other ARID family members. Last, other functional domains were not detected by protein database analysis using SMART [35] . We have recently identified Arid5a as a Sox9 co-regulator that promotes chondrogenesis through stimulating histone acetylation [28] . Histone acetylation is also important for gene transcription but is both functionally and structurally distinct from histone methylation, suggesting that Arid5a and Arid5b have distinct molecular functions. Pull-down assays demonstrated that Arid5a does not physically interact with Phf2, providing further evidence for the distinct functions of Arid5a and Arid5b ( Supplementary Fig. S9 ). Moreover, other regions besides the ARID domain of Arid5b and Arid5a are not conserved, which is why the Sox9-binding region of Arid5a is different from that of Arid5b. These data also suggest that Arid5b functions as an adaptor, forming a transcriptional complex with other transcriptional components using its unique C-terminal region to coordinate gene expression. In support of this, while several other ARID family members contain both jmjC and ARID domains in a single molecule, Arid5b includes only an ARID domain, and Phf2 includes only a jmjC domain [36] , [37] . This strongly implies that complex formation is required for the chondrogenic function of Arid5b. Our results showed that Sox9 physically bound the C terminus of Arid5b, and Baba et al . [27] demonstrated that the N terminus is responsible for the physical interaction between Arid5b and Phf2. Interestingly, the Arid5b (307–432) mutant that only comprises the ARID domain inhibited chondrogenesis both in vitro and in vivo . This is likely because this mutant can still bind to the Arid5b-binding element in promoters, but cannot associate with transcription factors such as Sox9. Therefore, this failure to assemble transcriptional complexes at these promoters leads to its dominant negative activity. Further investigation of additional Arid5b-interacting proteins will be important to gain further molecular insights into chondrocyte differentiation. In addition to chondrogenesis, several reports have shown that Arid5b is involved in mesenchymal cell differentiation. Arid5b promotes adipocyte differentiation of 3T3-L1 preadipocytic cell line, and MEFs isolated from Arid5b-deficient mice showed impaired adipogenesis [26] , [38] , [39] . It has also been reported that the expression of Arid5b is highly induced during the differentiation of MONC-1 cells into smooth muscle cells [40] , although H3K9me2 levels of the Myogenin promoter were not affected by Arid5b in C3H10T1/2 cells used in this study. As smooth muscle cells and adipocytes both originate from mesenchymal stem cells, Arid5b is likely to have important roles in the epigenetic regulation of mesenchymal cell differentiation. Moreover, we found that Arid5b was expressed in Sertoli cells in the testis ( Supplementary Fig. S2 ). Previous studies have indicated that the development of the testis, which is Sox9-dependent, is abnormal in Arid5b −/− mice [41] . These data collectively suggest that Arid5b has diverse functions in various tissues as a co-regulator for Sox9, as well as other transcription factors. Our results demonstrated that Arid5b induces chondrogenic gene expression through the recruitment of the histone demethylase Phf2, followed by demethylation of H3K9me2 in chondrogenic gene promoters. Histone modification by transcriptional co-regulators is an essential process for gene expression, and at least eight types of histone modification have been identified. However, to date, only the role of histone acetylation has been elucidated in chondrogenesis. Several groups have reported that Sox9 co-regulators directly or indirectly control histone acetylation coupled with chondrogenic gene expression [15] , [28] . However, recent progress in the epigenetic field has revealed that histone methylation/demethylation is a more upstream signal that is indispensable for dynamic gene activation and repression. There are likely more histone methyltransferases and demethylases than histone acetyltransferases and histone deacetylases, suggesting the greater importance of histone methylation in regulating gene expression [22] , [23] . Moreover, aberrant histone methylation has been linked to cellular differentiation and human disease, most prominently in cancer [42] , [43] . Despite their significance in gene expression, only a few groups have documented the involvement of histone methylation/demethylation in chondrocyte homoeostasis in adults [44] . Therefore, our findings provide new insights into the molecular mechanisms regulating endochondral ossification during skeletal development. The observation that Arid5b recruits the demethylase Phf2 to chondrogenic gene promoters indicates that H3K9me2 is an important signal for chondrocyte differentiation. H3K9 methylation is a highly conserved histone post-translational modification, and is highly linked with transcriptional repression. However, several studies have indicated that H3K9 is not the only methylated residue, and that the interplay between histone methylation and gene activation is complicated. Methylation at H3K4 and H3K36 activates gene expression, whereas H3K9 and H3K27 methylation appears to repress gene expression [22] , [23] . These reports indicate that various histone demethylases and/or methyltransferases might also associate with Sox9-dependent transcriptional complexes and help to regulate chondrogenic gene expression. As the final combination of histone modifications and their crosstalk determines the transcriptional outcomes in a spatiotemporal manner [45] , further studies are needed to clarify how histone modification controls chondrocyte differentiation. Although we show that Arid5b and Sox9 physically associate ( Fig. 2e ), as do Arid5b and Phf2 ( Fig. 5a ), we could not detect an interaction between Sox9 and Phf2. One possibility is that the interactions between the transcriptional complex components are dynamic, and many are transient and unstable. Gene expression is regulated at multiple steps, and different combinations of transcriptional co-regulators modulate each step. Thus, our findings may indicate that Arid5b sequentially regulates chondrocyte gene expression ( Supplementary Fig. S14 ). In this series of events, Arid5b would first form a complex with Phf2, and the complex would be recruited to chondrogenic gene promoters via the Arid5b-binding element. Second, Arid5b-associated Phf2 would stimulate the demethylation of H3K9me2 of these promoters. Third, the levels of H3K9me2 would increase the accessibility of Sox9 to the chondrogenic gene promoters. Finally, Sox9 and Arid5b would associate and cooperatively promote chondrogenesis. In conclusion, we have identified Arid5b as a transcriptional co-regulator for Sox9, which modulates chondrogenic gene expression through the regulation of histone demethylation. Our findings contribute to a more thorough understanding of the molecular mechanisms underlying Sox9-regulated chondrogenesis, and provide new insights into the epigenetic regulation of cartilage development. Cell culture and reagents NIH-3T3 cells and C3H10T1/2 cells were purchased from the RIKEN cell bank and cultured in Dulbecco’s Modified Eagle Medium (DMEM, Sigma-Aldrich, St Louis, MO, USA) containing 10% fetal bovine serum (FBS) at 37 °C in a humidified 5% CO 2 incubator. ATDC5 cells were purchased from the Riken cell bank and cultured in a 1:1 mixture of DMEM and Ham’s F-12 medium (Sigma-Aldrich) containing 10% FBS. Recombinant BMP2 was obtained from the conditioned media of CHO-K1 cells infected with BMP2 adenovirus [46] . The activity of BMP2 was determined by a comparison with human recombinant BMP2. Solexa deep sequencing Total RNA was isolated from NIH-3T3 cells and C3H10T1/2 cells using a total RNA isolation system (NucleoSpin RNAII, Macherey-Nagle, Duren, Germany). cDNA was synthesized using random hexamer primers and subjected to Solexa sequencing according to the manufacturer’s protocol. All tags were annotated using a database provided by Illumina. Real-time RT–PCR Total RNA was isolated using a total RNA isolation kit (Macherey-Nagel). After denaturation of total RNA at 70 °C for 10 min, cDNA was synthesized with oligo dT primers and reverse transcriptase (Takara, Shiga, Japan). Real-time RT–PCR amplification was performed using the TaqMan PCR protocol and the ABI 7300 real-time PCR system (Applied Biosystems, Carlsbad, CA, USA). The expression of Phf2 was quantified by real-time RT–PCR using SYBR Green . Primers and TaqMan probes used for amplification are listed in Supplementary Table S1 . The expression level of the mRNA was normalized by β-actin mRNA expression. Data are represented as mean±s.d. ( n =3). Western blotting Cells were rinsed twice with phosphate-buffered saline (PBS) and solubilized in lysis buffer (20 mM HEPES (pH 7.4), 150 mM NaCl, 1 mM EGTA, 1.5 mM MgCl 2 , 10% glycerol, 1% Triton X-100, 10 μg ml −1 aprotinin, 10 μg ml −1 leupeptin, 1 mM 4-(2-aminoethyl) benzenesulfonyl fluoride hydrochloride, 0.2 mM sodium orthovanadate). The lysates were centrifuged for 10 min at 4 °C at 15,000 g and boiled in sodium dodecyl sulphate (SDS) sample buffer containing 0.5 M β-mercaptoethanol for 5 min. The supernatant was separated by SDS–polyacrylamide gel electrophoresis (SDS–PAGE), transferred to nitrocellulose membranes, immunoblotted with primary antibodies and visualized with horseradish peroxidase-coupled anti-mouse or -rabbit immunoglobulin IgG antibodies using enhanced chemiluminescence detection kits (GE Healthcare, Buckinghamshire, UK). Anti-Arid5b (HPA015073, 1:500), anti-Flag (F3165, 1:10,000) and anti-Sox9 (AV37986, 1:1,000) antibodies were purchased from Sigma-Aldrich. Anti-HA (Y-11, 1:200), anti-Myc (9E-10, 1:200) and anti-β-actin (C4, 1:1,000) antibodies were purchased from Santa Cruz Biotechnology (Santa Cruz, CA, USA). The anti-Phf2 antibody was purchased from Cell Signaling Technology Japan (Tokyo, Japan). Full scans of western blotting data are listed in Supplementary Fig. S15 . Whole-mount in situ hybridization Digoxigenin-labelled antisense RNA probes were generated with SP6 or T7 RNA polymerase using the DIG RNA Labelling kit (Roche, Basel, Switzerland) according to the manufacturer’s instructions. Briefly, a DNA fragment of Arid5b (nucleotide positions, 1341–2075) was amplified by PCR and subcloned into a pCR2 TOPO vector (Invitrogen, Carlsbad, CA, USA). Plasmids containing Col2a1 and Sox9 fragments were kindly provided by Dr Toshihisa Komori (Nagasaki University Dental School, Nagasaki, Japan). C57BL/6 mouse embryos (E12.5) were fixed in 4% paraformaldehyde (PFA) in PBS overnight at 4 °C, and samples were then hybridized with gene-specific digoxigenin-labelled RNA probes at 70 °C overnight before being washed and incubated with anti-digoxigenin antibody (Anti-digoxigenin-AP, Roche). NBT (Nitroblue tetrazolium) and BCIP (5-bromo-4-chloro-3-indolyl phosphate p-toluidine) were used for signal detection. Immunohistochemistry Samples were fixed with 4% PFA–PBS, embedded in paraffin and cut into 5-μm-thick sections. They were then deparaffinized and stained with Mayer’s hematoxylin and eosin (H&E). Immunohistochemistry was performed using the following antibodies: anti-Col2 (#7050; Chondrex, Redmond, WA, USA) at a 1:500 (vol/vol) dilution and anti-Arid5b (NBP1-83622; Novus Biologicals, Littleton, CO, USA) at a 1:50 (vol/vol) dilution. Immunoreactivity was visualized with a biotinylated anti-rabbit IgG secondary antibody using the ABC Vectastain kit (Vector Laboratories, Burlingame, CA, USA) and the peroxidase substrate DAB kit (Vector Laboratories), according to the manufacturer’s protocol. Construction of expression vectors and transfection WT and mutants of Arid5b were amplified by PCR and subcloned into the Eco RI and Xba I sites of an expression vector containing a 6 × Myc, Flag, 3 × Flag or Venus epitope. Primer pairs used for PCR are as follows: 1–307: sense primer: 5′-GAATTCGAGCCCAACTCACTCCAGTGG-3′, antisense primer: 5′-ATCTAGATTATTCTTCATTTGAGACTTTTTT-3′; 307–432: sense primer: 5′-GAATTCAAACCAAAGGTTGCCATTGGT-3′, antisense primer: 5′-ATCTAGATTAATTTTCCTGTGAACTGTTCTC-3′; 432–1188: sense primer: 5′-GAATTCGAGAACAAAACAAAAGTATCT-3′, antisense primer: 5′-ATCTAGATTAACAGTTTTGTACTGGGGTGCAC-3′. Venus cDNA was kindly provided by Dr Atsushi Miyawaki (Riken). RFP-tagged Arid5b was generated by subcloning into pTurbo RFP-C (Evrogen, Moscow, Russia). Flag-tagged Phf2 was a kind gift from Dr Shigeaki Kato (The University of Tokyo). The WT and dominant negative mutant of Sox9 (a.a. 21–234) were amplified by PCR and subcloned into the Eco RI and Xba I sites of an expression vector containing an HA epitope [30] . Transfection of the expression vectors was carried out using FuGENE6 (Roche) according to the manufacturer’s protocol. Reporter assays A firefly luciferase reporter construct containing the human Col2a1 promoter (−89 to +16) and four 48-base pair tandem-repeats of the Sox9-binding element present in the first intron of the Col2a1 gene [47] were co-transfected with expression vectors into cells using the FuGENE6 reagent. After 48 h of transfection, the cells were lysed and luciferase activity was measured using specific substrates in a luminometer (Promega, Fitchburg, WI, USA) according to the manufacturer’s protocol. In vitro binding assays using His-tagged Sox9 and Arid5b The amplicon containing the coding region of Sox9 was subcloned into a pCold1 vector (Takara). The construct was transformed into the BL21 Escherichia coli strain and then His-tagged Sox9 protein expression was induced with isopropyl β-D-1-thiogalactopyranoside, and subsequently purified with Ni-NTA magnetic beads (QIAGEN, Venlo, The Netherlands) according to the manufacturer’s protocol. The purified His-tagged Sox9 protein was incubated with 293FT cell lysates transfected with 3 × Flag-tagged WT and mutant Arid5b. The association of Sox9 with Arid5b was determined by immunoblotting with an anti-Flag antibody. DNA pull-down assays Cells were lysed in lysis buffer (20 mM HEPES (pH 7.4), 150 mM NaCl, 1 mM EGTA, 1.5 mM MgCl 2 , 10% glycerol, 1% Triton X-100, 10 μg ml −1 leupeptin, 1 mM phenylmethanesulfonyl fluoride, 0.2 mM sodium orthovanadate). The lysates were pre-incubated with streptavidin agarose beads, then incubated for 3 h with 1 μg of a biotinylated double-stranded oligonucleotide probe that contained the Arid5b-binding element present in the Col2a1 promoter (sense primer: 5′-AAAGGGGCCGGGCGCATATAACGGGCGCCGCGGCGG-3′; antisense primer: 5′-CCGCCGCGGCGCCCGTTATATGCGCCCGGCCCCTTT-3′). Precipitated oligonucleotides were collected with Streptavidin magnetic beads (Dynabeads My One Streptavidin T1, Invitrogen) and washed with lysis buffer. Magnetic beads were resuspended with SDS-sample buffer, boiled for 5 min and subjected to western blot analysis. ChIP assays ChIP analysis was performed using a ChIP assay kit (ChIP-IT Express; Active Motif, Carlsbad, CA, USA) according to the manufacturer’s instructions. Briefly, C3H10T1/2 cells infected with Arid5b adenovirus or primary chondrocytes were washed with PBS, and the chromatin was fixed with 1% PFA. Chromatin shearing was performed using sonication. Chromatin was prepared and immunoprecipitated with anti-GFP and anti-H3K9me2 antibodies (Abcam, Cambridge, UK). An antibody against Phf2 was kindly provided by Dr Yuuki Imai (Ehime University, Matsuyama, Japan) [48] . The DNA fragments were precipitated with protein-A magnetic beads and amplified by PCR using primer pairs specific to the Col2a1 promoter containing the Arid5b-binding element (sense primer: 5′-GCGGGGTCTCAGGTTACAG-3′; antisense primer: 5′-GGTCTCTACCGCTCCCTCAT-3′). Quantitative analysis of ChIP assays was performed with real-time PCR; the primer pairs for ChIP real-time PCR are listed in Supplementary Table S2 . Arid5b-deficient mice To generate Arid5b-deficient mice, exon V of Arid5b was replaced with a neomycin resistance cassette (Neo r ) via homologous recombination [26] . Exon V encodes the third and fourth helices of the ARID structure, which lie in its hydrophobic core, and loss of Exon V disrupts the Arid structure [26] . The targeting vector was introduced via electroporation into ES cells derived from the 129S1 mouse strain. Arid5b heterozygous mice were backcrossed to a C57BL/6 background for >10 generations. To determine mouse genotypes, genomic DNA was PCR-amplified using the sense primer 5′-TGCATAGAATGAATGACCCTGGTC-3′ and the antisense primer 5′-CGGAAGTGGACAGATGG-AATGG-3′. The WT gene yields an 878-bp product and the Arid5b-deficient gene yields a 1,816 bp product. All experiments were performed with both male and female E15.5, P0 and 3-week-old littermate mice under protocols approved by Osaka University Graduate School of Dentistry animal committee. In situ hybridization Tibias from C57BL/6 mouse embryos (E14.5) were fixed in 4% PFA–PBS overnight at 4 °C, embedded in paraffin and cut into 5-μm sections. Digoxigenin-11-UTP-labelled single-stranded RNA probes were prepared using a DIG RNA labelling kit (Roche) according to the manufacturer’s instructions. We used a 0.4-kb fragment of mouse Col2a1 cDNA, a 0.65-kb fragment of mouse Col10a1 cDNA, a 0.57-kb fragment of mouse Ihh cDNA and a 0.8-kb fragment of mouse Pthr1 cDNA to generate antisense and sense probes. The signals were detected with alkaline phosphatase-conjugated anti-DIG antibody (Roche). All probes were kindly provided by Dr Noriyuki Tsumaki (Kyoto University, Kyoto, Japan) and Toshihisa Komori (Nagasaki University Dental School, Nagasaki, Japan). Knockdown of Phf2 siRNA for mPHF2 (siPhf2) (sense: 5′-CAGCAAACCUGACUCGUUAUU-3′, antisense: 5′-UAACGAGUCAGGUUUGCUGUU-3′) and control siRNA (siNC) were designed and purchased from Sigma-Aldrich. siRNA was introduced into primary chondrocytes using Lipofectamine RNAiMAX reagents (Life Technologies, Tokyo, Japan) according to the manufacturer’s protocol. Knockdown of endogenous Phf2 and its effects were examined 72 h after transfection. Statistical analysis The data were statistically analysed by Student’s t- test for two groups. For more than two groups, we used a one-way ANOVA or two-way ANOVA followed by the Tukey–Kramer test. P -values <0.05 were considered significantly different. Accession codes: Solexa deep sequencing data have been deposited in the DNA Data Bank of Japan ( http://www.ddbj.nig.ac.jp/ ) under accession number DRA001163 . How to cite this article: Hata, K. et al. Arid5b facilitates chondrogenesis by recruiting the histone demethylase Phf2 to Sox9-regulated genes. Nat. Commun. 4:2850 doi: 10.1038/ncomms3850 (2013).